Molecular mechanism for the control of virulentToxoplasma gondiiinfections in wild-derived mice Some strains of the protozoan parasite Toxoplasma gondii (such as RH) are virulent in laboratory mice because they are not restricted by the Immunity-Related GTPase (IRG) resistance system in these mouse strains. In some wild-derived Eurasian mice (such as CIM) on the other hand, polymorphic IRG proteins inhibit the replication of such virulent T. gondii strains. Here we show that this resistance is due to direct binding of the IRG protein Irgb2-b1 CIM to the T. gondii virulence effector ROP5 isoform B. The Irgb2-b1 interface of this interaction is highly polymorphic and under positive selection. South American T. gondii strains are virulent even in wild-derived Eurasian mice. We were able to demonstrate that this difference in virulence is due to polymorphic ROP5 isoforms that are not targeted by Irgb2-b1 CIM , indicating co-adaptation of host cell resistance GTPases and T. gondii virulence effectors. In the co-evolutionary process of host–pathogen interaction, adaptation to local conditions is critical. Infectious agents are a constant threat to multicellular organisms, and all metazoan organisms have evolved immune defense mechanisms to combat virulent microbes. Immune defense mechanisms emerge from selective pressures that microbes impose; invasive microbes, in turn, evolve to avoid or counteract immune effector mechanisms long enough to allow for efficient transmission. The host and the pathogen undergo co-adaptation at the molecular level. These equilibria are unstable and their conditions vary locally. Toxoplasma gondii is an obligate intracellular protozoan parasite belonging to the phylum Apicomplexa. It is distantly related to the genus Plasmodium , the causative agent of malaria. Unlike Plasmodium , however, T. gondii has an extraordinarily broad host range, with all true cats (Felidae) as definitive hosts and all warm-blooded animals, including birds and humans, as intermediate hosts. About one-fourth of the human population is infected with T. gondii , although local rates vary considerably [1] . A few lineages predominate in Europe and North America [2] , [3] , [4] and these canonical strains differ markedly in virulence in laboratory strains of mice. Virulent strains (e.g., restriction fragment length polymorphism (RFLP) genotype 10, previously called type I) are usually lethal following inoculation with even a single parasite, whereas the LD 50 (lethal dose, 50%) of avirulent strains (e.g., RFLP genoptypes 1, 2, 3, previously called types II and III) ranges between 10 3 and 10 5 in laboratory mice [5] , [6] . These virulence differences are due to a small number of polymorphic genes within the parasite genomes [7] , [8] , [9] . However, in other parts of the world, genetically highly diverse T. gondii strains have been isolated [4] , [10] , [11] , [12] , [13] , [14] , and especially in South America the majority of isolates is associated with high mortality rates in laboratory mice [11] , [15] . Immunity-Related GTPases (IRG) drive an essential mechanism of early cell-autonomous resistance against intracellular pathogens in mice [16] . IRG proteins are represented by about 20 single coding units in the C57BL/6 (BL/6) mouse genome [17] and multiple members are highly inducible by interferon-γ (IFNγ) [18] , [19] , [20] . The typical IRG gene has one or two short 5’-untranslated exons followed by a single long exon encoding the entire open reading fame. Four IRG genes depart from this structure, with two adjacent long exons each encoding a full-length IRG polypeptide, resulting in expression of proteins carrying two IRG domains joined by a short linker, subtending a single promoter, the so-called tandem IRG proteins [17] , [21] . Knockout (ko) mouse strains lacking single or multiple IRG members have consistently shown higher susceptibility to infection with normally avirulent T. gondii strains [22] , [23] , [24] . Following infection of an IFNγ-stimulated cell of a laboratory mouse, guanosine triphosphate (GTP)-activated effector IRG proteins begin to accumulate at the T. gondii parasitophorous vacuolar membrane (PVM) within minutes after invasion [25] , [26] , [27] . Premature activation in uninfected cells is prevented by the three regulator IRG proteins, Irgm1, 2 and 3, which keep the effector IRG proteins in a guanosine diphosphate (GDP)-bound inactive conformation at endogenous cellular membranes [28] , [29] until infection. The loading of effector IRG proteins is cooperative and hierarchical, with two family members serving as pioneers for members loading later in the hierarchy [26] . IRG protein accumulation is a prerequisite for subsequent disruption of the PVM [27] , [30] , [31] , [32] , which is in turn invariably followed by death of the parasite and subsequent necrotic death of the host cell [33] . A mechanochemical effector function of IRG proteins is suggested, by analogy to the dynamins [19] , [34] , to be responsible for the ruffling, vesiculation and ultimately disruption of the PVM observed at the microscopic level [27] , [30] , [32] . Virulence of T. gondii can be directly correlated with inactivation of the IRG resistance system. The initial loading of the PVM with IRG proteins is markedly reduced in virulent compared with avirulent strains [26] . To preserve the integrity of the PVM, T. gondii has evolved several polymorphic virulence effectors that are injected from secretory organelles (rhoptries and dense granules) directly into the cytosol during and after host cell invasion [1] , [35] . Genetic screens showed that the polymorphism in the rhoptry-derived ROP5 and ROP18 components of a secreted threonine kinase complex accounts for the differences in virulence between T. gondii strains in infected laboratory mice [5] , [36] , [37] . Several T. gondii effectors have been shown to inactivate mouse effector IRG proteins, thus preserving integrity of the PVM [38] , [39] , [40] , [41] , [42] , [43] , [44] , [45] . Recently, we showed considerable polymorphism in IRG proteins among several wild and wild-derived inbred mouse strains. The wild-derived Mus musculus castaneus strain CIM from South India counters effectors of Eurasian virulent strains, leading to encystment, and therefore potential transmission, of virulent parasites. In breeding experiments the resistance of CIM mice could be mapped to highly polymorphic IRG genes located on chromosome 11. Within this locus, one of the most polymorphic family members is the tandem IRG protein Irgb2-b1. We could show that in transiently transfected BL/6 cells, overexpression of Irgb2-b1 CIM can rescue the effector IRG protein, Irga6 BL/6 , from ROP5/ROP18/GRA7-mediated phosphorylation [21] . However, these observations did not show that protection of Irga6 is sufficient to enable wild-derived CIM mice themselves to fully resist infection by T. gondii virulent strains. Indeed, in BL/6 mice, resistance is only partially lost after deletion of Irga6 BL/6 [23] , suggesting that in the case of CIM mice, protection of Irga6 CIM by Irgb2-b1 CIM may not be sufficient to explain full resistance against virulent Eurasian T. gondii strains. In the present study, we show that Irgb2-b1 CIM is the CIM-inherited element largely responsible for resistance against virulent Eurasian T. gondii strains. We demonstrate efficient binding of Irgb2-b1 CIM only to virulent T. gondii -derived ROP5B but not ROP5A and ROP5C. The interface necessary for ROP5B binding is located within the N-terminal portion of Irgb2-b1 CIM and encompasses structural motifs that were previously shown to be under positive selection. Our findings are consistent with critical responsibility of ROP5 for the heightened virulence of T. gondii type I strains against laboratory Mus musculus , and inevitably suggest that other ROP pseudokinases may not play a significant role in virulence/avirulence behavior in mice against T. gondii . Furthermore, and supporting this last contention, we provide evidence that virulence of T. gondii strains from South America in CIM mice is due to a mismatch between Irgb2-b1 CIM and ROP5 isoforms. These results provide further evidence that T. gondii virulence and mouse resistance follow some form of allele-matching evolutionary dynamics. Irgb2-b1 CIM protects from virulent T. gondii strain infections Our own recent work demonstrates that the highly polymorphic Irgb2-b1 CIM tandem gene may be responsible for resistance of wild-derived CIM mice against virulent Eurasian T. gondii strains [21] . In transiently transfected IFNγ-induced BL/6 cells, expression of Irgb2-b1 CIM protected endogenous Irga6 BL/6 from ROP5/ROP18/GRA7-mediated phosphorylation by the virulent strain RH. High levels of Irgb2-b1 CIM at the PVM of T. gondii virulent strains were accompanied by absence of Irga6 BL/6 phosphorylation [21] . To test definitively the relevance of Irgb2-b1 CIM for the resistance of CIM cells against virulent T. gondii , we generated two independent lines of Irgb2-b1 CIM ko cells (T17 and i3) by CRISPR/Cas9 (clustered regularly interspaced short palindromic repeats/CRISPR-associated protein 9) nickase technology [46] . Loss of Irgb2-b1 CIM was confirmed in lysates of IFNγ-stimulated cells by western blot with an antibody specific for the C terminus of tandem IRG proteins (Fig. 1a ) [21] and Irgb2-b1 CIM could not be detected by immunofluorescence on vacuoles of RHΔ hxgprt strain T. gondii in ko cells (Fig. 1b , representative images are shown in Supplementary Fig. 1 ). Expression levels of IRG effector proteins Irga6, Irgb6, Irgb10 and Irgd, necessary for full resistance against avirulent strains of T. gondii in laboratory mice [16] , were not found to be different in CIM wild-type (wt) cells compared with Irgb2-b1 CIM ko cells (Fig. 1a ). Fig. 1 Irgb2-b1 CIM is largely responsible for resistance against virulent T. gondii strains. a Western blot of detergent lysates from CIM wild-type (wt) and Irgb2-b1 CIM knockout (ko) diaphragm-derived cells (DDCs) (T17 and i3) stimulated for 24 h with 200 U ml −1 interferon-γ (IFNγ). The signal representing Irgb2-b1 CIM in wt cells is lost in both ko cell lines (upper panel). Expression levels of all other Immunity-Related GTPases (IRG) proteins are unchanged in ko cell lines compared with wt cells (middle panels). Actin serves as loading control (lower panel). b , c Frequency of vacuoles positive for Irgb2-b1 CIM ( b ) or Irga6 CIM phosphorylated at T108 p(T108)Irga6 CIM ) ( c ) detected by immunofluorescence with anti-p(T108)Irga6 CIM or anti-Irgb2-b1 CIM antibodies in IFNγ-induced (200 U ml −1 ) wt CIM and BL/6 or Irgb2-b1 CIM ko CIM DDCs infected for 2 h with RHΔ hxgprt . Error bars indicate the mean and standard error of the mean (SEM) of three ( b ) or four ( c ) independent experiments (about 100 vacuoles were counted per experiment). One-way analysis of variance (ANOVA) followed by Tukey's multiple comparison was used to test differences between groups; **** p < 0.0001; ** p < 0.0025; n.s. not significant. b No Irgb2-b1 CIM positive vacuoles were found in Irgb2-b1 CIM ko cells. c Frequencies of p(T108)Irga6 CIM -positive vacuoles in ko cells are significantly increased in comparison with wt cells. d , e CIM DDCs were induced with 100 U ml −1 IFNγ for 24 h and infected with T. gondii RH-YFP at a multiplicity of infection (MOI) of 1 or 3. Intracellular parasite growth was determined by flow cytometry 24 h post infection as described in Methods. Error bars indicate the mean and SEM of three independent experiments. One-way ANOVA followed by Tukey's multiple comparison was used to test differences between groups; **** p < 0.0001; n.s. not significant. d Control of T. gondii replication is lost in wt BL/6 and Irgb2-b1 CIM ko CIM DDCs compared with wt CIM DDCs. e Control of T. gondii replication is restored to wt levels (wt CIM DDCs) in Irgb2-b1 CIM ko CIM DDCs complemented with Irgb2-b1 CIM (T17+Irgb2-b1 CIM ) Full size image Phosphorylation of Irga6 BL/6 in susceptible BL/6 cells by the ROP5/ROP18/GRA7 kinase complex of virulent T. gondii strains occurs mainly at two threonine residues (T102 and T108) in the G-domain [39] , [40] . In wt CIM cells, Irga6 CIM phosphorylation by RHΔ hxgprt strain T. gondii is almost completely inhibited (Fig. 1c ); however, in the two Irgb2-b1 CIM ko CIM cell lines, the frequencies of vacuoles carrying pT108-phosphorylated Irga6 CIM are comparable to frequencies in BL/6 cells (Fig. 1c , representative images are shown in Supplementary Fig. 2 ). The ability of IFNγ-induced CIM wt and Irgb2-b1 CIM ko cells to control replication of RH-YFP was compared in infected cells by flow cytometry (Fig. 1d , gating strategy and representative images are shown in Supplementary Fig. 3 ) and incorporation of 3 H-uracil (Supplementary Fig. 4 ). In both assays, Irgb2-b1 CIM ko cells lost the ability to restrict T. gondii virulent strain replication shown by CIM wt cells. The Irgb2-b1 CIM ko cell line T17 was complemented with Irgb2-b1 CIM and Irgb2-b1 CIM expression was confirmed by western blot of detergent lysates (Supplementary Fig. 5 ). In unstimulated cells, Irgb2-b1 CIM expression is only detectable in complemented but not wt cells (left hand panel), whereas upon stimulation with IFNγ, Irgb2-b1 CIM levels are similar in CIM wt and complemented cells (right hand panel). Low Irgb2-b1 expression levels in BL/6 wt cells have been described earlier [21] , and Irgb2-b1 CIM ko cells show no signs of Irgb2-b1 CIM expression. Complementation of ko cells with Irgb2-b1 CIM restored resistance against virulent T. gondii RH-YFP to wt levels (Fig. 1e ). Irgb2-b1 CIM is mainly associated with ROP5B Several published results have demonstrated a specific molecular interaction between the ROP5 pseudokinase component of the ROP5/ROP18/GRA7 kinase complex of virulent Eurasian T. gondii strains, and the IRG effector, Irga6 BL/6 [38] , [41] , [43] , [47] . A structurally similar interaction has been proposed between Irgb2-b1 CIM and ROP5 based on the predicted architecture shared by all IRG proteins [48] . In contrast to other IRG proteins, ROP5 of the mouse virulent strain RH is required for vacuolar loading of Irgb2-b1 CIM and variation in ROP5 expression levels of different T. gondii RH sub-strains correlate directly with the amount of vacuolar Irgb2-b1 CIM loading. In CIM cells, vacuoles of rop5 -deficient RH load very little Irgb2-b1 CIM [21] . A plausible explanation is that virulent ROP5 bound to the vacuolar membrane is a direct target for Irgb2-b1 CIM . We here demonstrate an Irgb2-b1 CIM /ROP5 interaction by co-immunoprecipitation from detergent lysates of CIM cells infected with the T. gondii virulent RHΔ hxgprt strain (Fig. 2a , upper left hand panel). Protein amounts in the lysates used for co-immunoprecipitation are shown in the middle and right hand panels. This interaction could be confirmed by pull-down of ROP5 from T. gondii tachyzoite detergent lysates with a purified Irgb2-b1 CIM glutathione S -transferase (GST)-fusion protein. When the BL/6 variant of Irgb2-b1 was used, no binding to ROP5 was detectable under similar conditions (Fig. 2b , middle left hand panel). Equal protein amounts and validation of T. gondii strains used in the pull-down were confirmed with tachyzoite lysates (Fig. 2b , right hand panels). In both experiments (Fig. 2a, b ) appearance of GRA7 in the pull-down is consistent with a direct interaction with ROP5, as previously demonstrated [43] . Fig. 2 Irgb2-b1 CIM directly binds T. gondii -derived ROP5B and ROP5C. a Irgb2-b1 CIM was co-imunoprecipitated from RHΔ hxgprt - but not RHΔ rop5 -infected CIM diaphragm-derived cells (DDCs) that have been induced with 200 U ml −1 interferon-γ (IFNγ) using a ROP5-specific antibody (upper left hand panel). The lower left hand panel indicates GRA7 association with ROP5 immunoprecipitations. The star indicates a protein unspecifically detected by the antibody used for immunoprecipitation. The middle and right hand panels display amounts of ROP5, GRA7 and Irgb2-b1 in the lysates used for immunoprecipitation. b Pull-down of ROP5 by CIM but not BL/6 GST-Irgb2-b1 from RHΔ hxgprt detergent lysates. RHΔ rop5 tachyzoite detergent lysates have been included as control (middle left hand panel). The lower panel indicates GRA7 association with ROP5. The upper panel indicates input of glutathione S -transferase (GST)-fusion proteins in the pull-down. The right hand blot shows ROP5 (upper panel) and GRA7 (lower panel) levels in tachyzoite lysates. c Irgb2-b1 CIM interacts with ROP5B and ROP5C but not ROP5A in a yeast two-hybrid approach. Proteins were expressed either as fusion to a transcriptional activation domain (AD) from pGAD-C3 or to a DNA-binding domain (BD) from pGBD-C3. Colony growth under 3DO conditions is indicative of protein/protein interaction. The bold black line separates samples from negative controls. d Protein-fragment complementation assay. Proteins were fused to N-terminal (BlaN) or C-terminal (BlaC) fragments of the reporter protein TEM - 1 β-lactamase. The increase in absorbance measured at 405 nm indicates restoration of β-lactamase activity after protein/protein interaction. Binding of Irgb2-b1 CIM to ROP5B is significantly stronger compared to ROP5C and ROP5A. Error bars indicate the mean and standard deviation of three independent experiments (right hand panel). One-way analysis of variance (ANOVA) followed by Tukey's multiple comparison was used to test differences between groups; **** p < 0.0001; ** p < 0.0025. The kinetic of the β-lactamase reaction is shown for one representative experiment (left hand panel) Full size image These data demonstrate that recruitment of Irgb2-b1 CIM to the PVM of T. gondii virulent RHΔ hxgprt strain is dependent on ROP5. However, they neither prove a direct binary interaction nor discriminate between distinctive ROP5 isoforms A, B and C. The yeast two-hybrid (Y2H) assay allows direct screening for interaction of two proteins. Therefore, Irgb2-b1 CIM and virulent RHΔ hxgprt T. gondii isoforms ROP5A/B/C were expressed as N-terminal fusion proteins with the Gal4 DNA-binding (BD) or Gal4 activation domain (AD) in a yeast reporter strain. Colony growth on selective medium indicated direct interaction of Irgb2-b1 CIM with ROP5B. Significantly less colony growth was observed for ROP5C, and no interaction with ROP5A was detectable (Fig. 2c ). In the protein-fragment complementation assay (PCA), binding of Irgb2-b1 CIM to ROP5 isoforms B and C could be reproduced and, also in this case, binding to ROP5B was significantly stronger than to ROP5C (Fig. 2d ). The Irgb2-b1 CIM interface for ROP5B binding is under positive selection Many IRG proteins are highly polymorphic in Mus musculus , but only the N-terminal unit of the Irgb2-b1 tandem, Irgb2, has been under recent positive selection [21] . A significant evolutionary hotspot encompassing putative structural motifs αd and H4 spans Irgb2 nucleotides 500 to 700. Both αd and H4 constitute essential parts of the Irga6 BL/6 interface for ROP5 binding [38] , [47] and we considered that these motifs probably also participate in Irgb2-b1 CIM binding to ROP5. Initially, the N-terminal moiety Irgb2 CIM and C-terminal moiety Irgb1 CIM were expressed separately as GST-fusion proteins and applied in a pull-down approach with T. gondii virulent tachyzoite detergent lysates. Binding of Irgb2 CIM but not Irgb1 CIM to T. gondii -derived ROP5 (Fig. 3a ) strongly suggests that the interface for ROP5 binding is located in the polymorphic N-terminal part of Irgb2-b1 CIM . Input of GST-fusion proteins (Fig. 3a , upper left hand panel) and protein amounts in the tachyzoite lysate used in the pull-down (Fig. 3a , right hand panels) is shown. To demonstrate that αd and H4 of Irgb2 CIM are responsible for ROP5 recognition, a chimeric Irgb2-b1 protein was generated and tested for ROP5 binding. The Irgb2-b1 Chimera encompasses a modified Irgb2 CIM , where αd and H4 were replaced with the respective BL/6 sequences, followed by full-length Irgb1 BL/6 (Fig. 3b ). Fig. 3 The Irgb2-b1 CIM interface for T. gondii ROP5B binding is polymorphic. a Pull-down of T. gondii ROP5 by GST-Irgb2 CIM but not GST-Irgb1 CIM from RHΔ hxgprt tachyzoite detergent lysates (lower left hand panel). The upper left hand panel indicates input of glutathione S -transferase (GST)-fusion proteins in the pull-down. The right hand panels display amounts of ROP5 (upper panel) and GRA7 (lower panel) in the tachyzoite lysate used for the pull-down. b Schematic representation of Irgb2-b1 CIM-BL/6 chimeric variant (Irgb2-b1 Chimera ) used in ( c , d ). c , d Irgb2-b1 CIM interaction with T. gondii ROP5B but not ROP5C is disturbed in case of Irgb2-b1 Chimera . c Protein-fragment complementation assay. Proteins were fused to N-terminal (BlaN) or C-terminal (BlaC) fragments of the reporter protein TEM - 1 β-lactamase. Error bars indicate the mean and standard deviation of three independent experiments (right hand panel). One-way analysis of variance (ANOVA) followed by Tukey's multiple comparison was used to test differences between groups; **** p < 0.0001; n.s. not significant. The kinetic of the β-lactamase reaction is shown for one representative experiment (left hand panel). Interaction of Irgb2-b1 CIM with T. gondii ROP5B is almost completely abrogated with Irgb2-b1 Chimera . d Yeast two-hybrid approach. Proteins were expressed either as fusion to a transcriptional activation domain (AD) from pGAD-C3 or to a DNA-binding domain (BD) from pGBD-C3. Colony growth under 3DO conditions is indicative of protein/protein interaction. Black dotted lines indicate assembly of relevant areas from two different plates. e Intensities of individual vacuoles positive for Irgb2-b1 CIM and Irgb2-b1 Chimera detected by immunofluorescence with anti-Irgb2-b1-specific antiserum in interferon-γ (IFNγ)-induced (200 U ml −1 ) wild-type (wt) CIM diaphragm-derived cells (DDCs) infected for 2 h with RHΔ hxgprt . Intensities of Irgb2-b1 Chimera are significantly reduced at RHΔ hxgprt -derived vacuoles. f Frequency of Irgb2-b1 CIM - and Irgb2-b1 Chimera -positive vacuoles detected by immunofluorescence with anti-Irgb2-b1-specific antiserum in IFNγ-induced (200 U ml −1 ) complemented Irgb2-b1 ko CIM DDCs infected for 2 h with RHΔ hxgprt (about 100 vacuoles were counted per experiment). No differences in numbers of Irgb2-b1 CIM - and Irgb2-b1 Chimera -positive vacuoles could be observed. In e and f , error bars indicate the mean and SEM of three independent experiments. Student's t-test was used for two-group comparisons; **** p < 0.0001, n.s. not significant Full size image In the PCA, binding of the Irgb2-b1 Chimera to ROP5B was almost completely abrogated, whereas binding to ROP5C was even more pronounced than wt Irgb2-b1 CIM binding to ROP5C (Fig. 3c ). These results were confirmed in a Y2H approach. Only ROP5C but not ROP5B binding to Irgb2-b1 Chimera could be observed (Fig. 3d ). Binding of Irgb2-b1 Chimera to ROP5C was also reflected in recruitment to the T. gondii virulent strain-derived PVM. After complementation of Irgb2-b1 CIM ko cells, the vacuolar intensities of Irgb2-b1 Chimera are significantly lower than Irgb2-b1 CIM , but still detectable (Fig. 3e ). We could not observe differences in numbers (protein intensities are not considered in these analyses) of Irgb2-b1 CIM - and Irgb2-b1 Chimera -positive vacuoles (Fig. 3f ) confirming the association of both proteins with different ROP5 isoforms. ROP5B is the main isoform responsible for T. gondii virulence in vitro Binding of Irgb2-b1 Chimera to ROP5C stimulated us to reinvestigate binding of Irgb2-b1 BL/6 to virulent strain-derived ROP5 isoforms. In the PCA, only binding of Irgb2-b1 BL/6 to ROP5C, but not to ROP5B or ROP5A, could be detected (Fig. 4a ); these results were further confirmed by Y2H analysis (Fig. 4b ). Surprisingly, Irgb2-b1 BL/6 binding to ROP5C could not be detected in the pull-down with a GST-tagged fusion protein (Fig. 2b ) but this proved to be due to discrimination between ROP5 isoforms by the antibody used in subsequent western blot analysis since, after overexpression of single FLAG-tagged ROP5 isoforms in transiently transfected cells, the anti-ROP5-specific antibody 3E2 detects ROP5A and ROP5B but not ROP5C in the western blot of detergent cell lysates. Protein expression was verified with an anti-FLAG antibody, with calnexin levels serving as loading control (Supplementary Fig. 6 ). Phylogenetic analysis of Irgb2 sequences [21] reveals the allelic diversity between laboratory and wild-derived mice (Fig. 4e , upper panel). An alignment of amino acids 167 to 233 encompassing putative structural motifs αd and H4 highlight the polymorphic residues within this region (Fig. 4e , lower panel). To confirm the different binding specificities for ROP5B in infected cells, we used RH∆ rop5 parasites expressing virulent allelic isoforms ROP5A and ROP5B with HA- or FLAG-epitope tag (RH∆ rop5 +A/B expressing HA-ROP5A and FLAG-ROP5B) [49] . We can demonstrate ROP5B binding to Irgb2-b1 CIM but not Irgb2-b1 BL/6 or Irgb2-b1 Chimera by co-immunoprecipitation from detergent lysates of cells infected with T. gondii RH∆ rop5 +A/B (Supplementary Fig. 7 ) again suggesting that residues within this polymorphic hotspot determine the interaction. Protein amounts in the lysates used for co-immunoprecipitation are shown (Supplementary Fig. 7 , middle and right hand panels). Fig. 4 Irgb2-b1 BL/6 directly binds ROP5C. a Protein-fragment complementation assay. Proteins were fused to N-terminal (BlaN) or C-terminal (BlaC) fragments of TEM - 1 β-lactamase. One-way analysis of variance (ANOVA) followed by Tukey's multiple comparison was used to test differences between groups; **** p < 0.0001; n.s. not significant. The kinetic of the reaction is shown for one representative experiment (left hand panel). Irgb2-b1 BL/6 interacts with T. gondii ROP5C but not ROP5B and ROP5A. b Yeast two-hybrid. Proteins were expressed as fusion with transcriptional activation domain (AD) from pGAD-C3 or DNA-binding domain (BD) from pGBD-C3. Colony growth is indicative of Irgb2-b1 BL/6 and Irgb2-b1 Chimera interaction with ROP5C and Irgb2-b1 CIM interaction with ROP5B. Bold black lines separate samples from negative controls. c Intensities of individual vacuoles detected by immunofluorescence with anti-Irgb2-b1-specific antiserum in interferon-γ (IFNγ)-induced (200 U ml −1 ) cells infected for 2 h with RHΔ hxgprt . Kruskal–Wallis test followed by Dunn's multiple comparisons was used to test differences between groups; **** p < 0.0001; n.s. not significant. Intensities of Irgb2-b1 BL/6 and Irgb2-b1 Chimera are reduced at RHΔ hxgprt -derived vacuoles. d Polymorphic Irgb2-b1 CIM interface mediating ROP5B binding is crucial for T. gondii control in vitro. CIM diaphragm-derived cells (DDCs) were induced with 100 U ml −1 IFNγ for 24 h and infected with T. gondii RH-YFP at a multiplicity of infection (MOI) of 1 or 3. Parasite growth was determined by flow cytometry 24 h post infection. One-way ANOVA followed by Dunnett's multiple comparisons was used to test differences between CIM wild-type (wt) and other cells; **** p < 0.0001; *** p < 0.0008; ** p < 0.006; n.s. not significant. Control of T. gondii virulent strain replication is lost in Irgb2-b1 CIM ko CIM DDCs complemented with Irgb2-b1 Chimera . e Upper panel, phylogenetic analysis and maximum likelihood tree of Irgb2 sequences (CIM, M. m. castaneus ; CAST, M. m. castaneus ; LAB, M. m. domesticus ; PWK, M. m. musculus ; SPRET, Mus spretus ). LAB indicates the allele shared by all laboratory mice tested so far, including C57BL/6 [21] . Only bootstrap values above 50 are shown. Lower panel, alignment of Irgb2 amino acids M167 to P233 encompassing putative structural motifs αd and H4. Polymorphic sites are highlighted in blue. Error bars indicate the mean and SEM or standard deviation of three independent experiments Full size image Irgb2-b1 BL/6 binding to ROP5C can account for the residual protein amounts at the PVM in T. gondii virulent strain-infected Irgb2-b1 CIM ko cells complemented with Irgb2-b1 BL/6 (Fig. 4c ). The possibility that Irgb2-b1 BL/6 and Irgb2-b1 Chimera interaction with ROP5C might contribute to parasite control was investigated by flow cytometry of infected cells. Expression of these particular proteins in Irgb2-b1 CIM ko cells did not result in increased growth inhibition of virulent T. gondii compared to CIM wt cells or Irgb2-b1 CIM ko cells complemented with Irgb2-b1 CIM (Fig. 4d ), suggesting that ROP5C does not contribute significantly to virulence of Eurasian T. gondii strains in CIM cells. T. gondii strains from South America are not restricted by Irgb2-b1 CIM T. gondii isolates from South America are genetically highly diverse, and the majority is associated with high mortality rates in laboratory mice. We compared virulence of T. gondii strains VAND and AS28, both originating from South America, in CIM mice. Unlike virulent Eurasian T. gondii strains [21] , VAND (Fig. 5a ) and AS28 (Fig. 5b ) are lethal in CIM mice. Fig. 5 South American T. gondii VAND and AS28 evade growth restriction in CIM mice. CIM wild-type (wt) ( a , n = 25; b , n = 19) and C57BL/6 ( a , n = 15; b , n = 10) mice were infected by intraperitoneal injection of 1000 T. gondii VAND ( a ) or 100 AS28 ( b ) strain parasites and survival monitored for 15–20 days. Data shown are combined from three ( a ) or two ( b ) independent experiments Full size image T. gondii VAND-derived ROP5 isoforms are not targeted by Irgb2-b1 CIM The first step to identify the molecular constituents that account for virulence of T. gondii strains from South America in CIM mice was to determine activity of the ROP5/ROP18/GRA7 kinase complex on Irga6 CIM . We assessed Irga6 CIM phosphorylation in T. gondii -infected CIM cells by immunfluorescence analysis. Mean p(T108)Irga6 CIM intensities were increased in CIM cells infected with T. gondii VAND, but not with AS28, compared with RHΔ hxgprt (Fig. 6a ). Since high p(T108)Irga6 levels have already been shown to correlate with low Irgb2-b1 intensities [21] , we considered the possibility that Irgb2-b1 CIM levels on VAND-derived vacuoles in CIM cells might be lower than on RHΔ hxgprt . This, in turn, would suggest that Irgb2-b1 CIM interacts inefficiently with ROP5 variants expressed by VAND. We therefore determined vacuolar Irgb2-b1 CIM intensities in T. gondii RHΔ hxgprt -, VAND- and AS28-infected CIM cells. Irgb2-b1 CIM intensities at vacuoles of both AS28 and VAND were clearly decreased relative to RHΔ hxgprt (Fig. 6b , representative images are shown in Supplementary Fig. 8 ). Indeed, in the case of VAND, Irgb2-b1 CIM levels were similar to those observed at vacuoles of RHΔ rop5 parasites [21] , suggesting that VAND ROP5 does not interact at all with Irgb2-b1 CIM. These results were confirmed in pull-down experiments from tachyzoite lysates with GST-tagged Irgb2-b1 CIM ; binding of Irgb2-b1 CIM to ROP5 was reduced in case of T. gondii AS28 and not detectable in case of T. gondii VAND (Fig. 6c ). Input of GST-Irgb2-b1 CIM (Fig. 6c , upper left hand panels) and protein amounts in the tachyzoite lysates used in the pull-down (Fig. 6c , right hand panels) is shown. These results correlate well with results obtained by immunofluorescence analysis (Fig. 6b ). Equal ROP5 expression levels and recognition of AS28 and VAND ROP5 variants by the anti-ROP5 antibody used for western blot analysis could be confirmed after immunoprecipitation from extracellular tachyzoite lysates (Supplementary Fig. 9 ). Recently we demonstrated that T. gondii GRA7 is associated with ROP5 [43] but surprisingly, VAND GRA7 was detected in the GST-Irgb2-b1 CIM pull-down in the absence of ROP5 binding (Fig. 6c ). This proved to be due to a direct interaction between VAND GRA7 and empty GST beads (Supplementary Fig. 10a ). Further evidence that GRA7 is not a functional inhibitor of VAND ROP5 association with Irgb2-b1 CIM was provided by Y2H analysis. Here, in the absence of VAND GRA7, none of the VAND ROP5 isoforms, ROP5A, B1, B2 and B3, interacted with Irgb2-b1 CIM (Fig. 6d ), suggesting that an intrinsic polymorphism of ROP5 VAND is responsible for its failure to interact with Irgb2-b1 CIM . Moreover, the YTH results confirm that absolute absence of ROP5 VAND binding to Irgb2-b1 after pull-down (Fig. 6c ) is not simply due to failure of the antibody used in the western blot to recognize ROP5 VAND isoforms. ROP5 uses a surface for binding to Irga6 BL/6 that is highly polymorphic and under positive selection [49] . When T. gondii RH and VAND rop5 alleles are compared, several amino acid substitutions within this region can be found [41] , [50] (Fig. 6e ). We created a ROP5B3 VAND mutant carrying the ROP5B RH interface for Irga6 BL/6 binding (ROP5B Chimera ) and investigated binding to Irgb2-b1 CIM . In the PCA assay, binding of ROP5B3 VAND to Irgb2-b1 CIM is significantly reduced compared to ROP5B Chimera and Irgb2-b1 CIM (Supplementary Fig. 11 ). Fig. 6 T. gondii VAND-derived ROP5 escapes targeting by Irgb2-b1 CIM . a p(T108)Irga6 CIM protein intensities are increased at VAND-derived vacuoles. interferon-γ (IFNγ)-induced CIM diaphragm-derived cells (DDCs; 200 U ml −1 ) were infected for 2 h with indicated T. gondii strains and individual p(T108)Irga6 CIM -positive vacuoles identified with 558 p(T108)Irga6 CIM -specific antiserum. Error bars indicate the mean and SEM of three independent experiments. Kruskal–Wallis test followed by Dunn's multiple comparisons was used to test differences between groups; **** p < 0.0001; n.s. not significant. b Irgb2-b1 CIM intensities are reduced at VAND- and AS28-derived vacuoles. IFNγ-induced CIM DDCs (200 U ml −1 ) were infected for 2 h with indicated T. gondii strains and individual Irgb2-b1 CIM -positive vacuoles identified with anti-Irgb2-b1-specific antiserum. Error bars indicate the mean and SEM of three independent experiments. Kruskal–Wallis test followed by Dunn's multiple comparisons was used to test differences between groups; **** p < 0.0001; ** p < 0.006. c In vitro pull-down with recombinant GST-Irgb2-b1 CIM fusion protein and T. gondii tachyzoite detergent lysates. Pull-down of ROP5 by Irgb2-b1 CIM is reduced with AS28 and completely lost in case of VAND tachyzoite lysates compared to RHΔ hxgprt -derived ROP5 (middle left hand panel). VAND GRA7 pull-down is not dependent on ROP5 (lower panel). The upper panel indicates input of GST-Irgb2-b1 CIM in the pull-down. The right hand blot shows ROP5 (upper panel) and GRA7 (lower panel) levels in tachyzoite lysates. All tracks were run on a single gel; vertical white lines indicate excision of irrelevant tracks. d VAND ROP5 isoforms ROP5A, ROP5B1, ROP5B2 and ROP5B3 do not directly interact with Irgb2-b1 CIM or VAND GRA7 in a yeast two-hybrid approach. Proteins were expressed either as fusion to a transcriptional activation domain (AD) from pGAD-C3 or to a DNA-binding domain (BD) from pGBD-C3. Colony growth under 3DO conditions is indicative of protein/protein interaction. Bold black line separates samples from negative controls. e Upper panel, alignment of T. gondii RH and VAND ROP5 amino acid sequences that represent a polymorphic hotspot and have been shown to be involved in binding to Irga6 BL/6 . Polymorphic sites are highlighted in blue. Lower panel, phylogenetic analysis and maximum likelihood tree of T. gondii RH and VAND rop5 sequences. Only maximum likelihood bootstrap values above 50 are shown Full size image Restriction of T. gondii growth in mice is dependent on IFNγ-inducible IRG and GBP (guanylate-binding protein) proteins that accumulate at the PVM leading to its rupture, death of the parasite and necrotic death of the host cell [16] , [51] . T. gondii virulent strains are able to overcome cell-autonomous resistance by secretion of effector proteins that inactivate IRG and GBP protein function [52] , [53] . Certain T. gondii strains of the RFLP genotype 10 (formerly type I) are highly virulent for laboratory mice but are well resisted in CIM wild-derived mice. In the latter, polymorphic IRG proteins on Chr11 were shown to protect CIM mice from T. gondii virulent strain infections and the highly polymorphic tandem IRG protein Irgb2-b1 CIM was implicated [21] . In this study, we have shown by gene deletion and complementation that polymorphic variation in Irgb2-b1 is indeed responsible for the restriction of virulent T. gondii strains in CIM cells and the failure of restriction in C57BL/6 (BL/6) cells (Fig. 7 ). Two independent Irgb2-b1 CIM ko CIM cell lines lost the ability to control T. gondii virulent strain replication compared to wt cells. Complementation of ko cells with Irgb2-b1 CIM restored resistance to wt levels (Fig. 1e ). Phosphorylation of Irga6 is a good indicator for parasite virulence [39] , [40] and loss of parasite control in the absence of Irgb2-b1 CIM is reflected in elevated numbers of p(T108)Irga6 CIM -positive vacuoles upon virulent strain infection (Fig. 1c ). Fig. 7 Model for Irgb2-b1-mediated control of T. gondii infection in wild-derived mice. a In laboratory mice, effector proteins from canonical virulent T. gondii strains (like RH) specifically phosphorylate certain Immunity-Related GTPases (IRG) proteins, thereby inhibiting oligomerisation and destruction of the parasitophorous vacuolar membrane (PVM). Two rhoptry kinases, ROP18 and ROP17, have been demonstrated to preferentially phosphorylate Irga6 BL/6 or Irgb6 BL/6 . The existence of additional parasite effectors specific for other IRG proteins is assumed. b In CIM and probably other wild-derived mice, canonical virulent T. gondii strains (like RH) are counteracted by direct binding of ROP5 isoform B by the polymorphic tandem IRG protein Irgb2-b1 CIM . IRG effector proteins are free to accumulate around the PVM, resulting in growth control, encystment and transmission of the parasite. Genetically more diverse T. gondii strains, like T. gondii VAND from South America, express polymorphic ROP5 variants that are not targeted by Irgb2-b1 CIM . Consequently, effector IRG proteins such as Irga6 CIM are phosphorylated and inactivated by a T. gondii VAND kinase complex. Infected animals die shortly after parasite challenge. Molecular interaction between ROP18 and ROP5 or Irga6 and ROP5 within the VAND kinase complex awaits experimental confirmation Full size image In our earlier study, overexpression of Irgb2-b1 CIM in transiently transfected BL/6 cells rescued endogenous Irga6 BL/6 from ROP5/ROP18/GRA7-mediated phosphorylation. In the same study Irgb2-b1 CIM was itself shown to be phosphorylated by virulent ROP5/ROP18 but this phosphorylation did not inhibit its PVM accumulation. Surprisingly and in stark contrast to other IRG proteins, vacuolar accumulation of Irgb2-b1 CIM is strictly dependent on T. gondii -derived ROP5; lower ROP5 levels correlate with decreased amounts of Irgb2-b1 CIM [21] . Based upon these results, we investigated binding of Irgb2-b1 CIM to ROP5 as the underlying molecular mechanism of CIM-inherent resistance. Here we demonstrate direct binding of Irgb2-b1 CIM to T. gondii -derived ROP5. The result provides corroborative evidence that Irgb2-b1 CIM traps ROP5, leading to diversion of the ROP18 kinase function from Irga6 to Irgb2-b1, and in that way confers cell-autonomous resistance against virulent T. gondii strains. Interestingly, binding of Irgb2-b1 CIM to ROP5 is isoform specific. The impact of ROP5 isoforms on T. gondii virulence has been investigated in former studies. Single or pair-wise combinations of rop5 isoforms were tested to rescue the virulence phenotype in RHΔ rop5 organisms. Complementation with one or two copies of rop5 A RH only partially rescued virulence and only rop5 A RH in combination with rop5 B RH displayed a phenotype indistinguishable from parental strain infections [49] . Otherwise, when ROP5A RH or ROP5C RH was expressed alone in a T. gondii avirulent genetic background, Irgb6 BL/6 loading was decreased compared to wt strain infections. However, none of these ROP5 isoforms increased parasite virulence in mice [41] . The effect of ROP5B RH alone on T. gondii virulence has never been investigated. In all our assays, efficient binding of Irgb2-b1 CIM could be observed only to ROP5B RH but not to ROP5C RH or ROP5A RH . Irgb2-b1 BL/6 was strongly associated with ROP5C RH ; the meaning of this unexpected result is not immediately clear since Irgb2-b1 BL/6 is expressed at very low levels in BL/6 cells. Furthermore, complementation of an Irgb2-b1 CIM ko cell line with Irgb2-b1 BL/6 does not confer resistance against T. gondii virulent strain infection. Certainly these findings indicate a predominant responsibility of ROP5B RH as opposed to the A or C isoforms for the virulence of virulent Eurasian T. gondii strains in laboratory mouse strains, and Irgb2-b1 CIM is its principal antagonist in CIM mice and presumably other strains that have the same Irgb2-b1 allele. Low expression levels of endogenous Irgb2-b1 BL/6 result in negligible numbers of Irgb2-b1 BL/6 -positive vacuoles of virulent T. gondii and correspondingly high virulence. However, the failure of Irgb2-b1 BL/6 , unlike Irgb2-b1 CIM , to attenuate virulence is due not only to its low expression level but also to its different amino acid sequence since overexpression of Irgb2-b1 BL/6 in BL/6 cells increases the number of Irgb2-b1 BL/6 -positive RHΔ hxgprt strain vacuoles (presumably this Irgb2-b1 BL/6 association with the PVM is due to binding to ROP5C (Fig. 4 )) but does not increase endogenous Irgb6 BL/6 loading [21] . Comparative sequence analysis suggested that so far the N-terminal unit, Irgb2, of the Irgb2-b1 tandem is the only IRG sequence that is under recent divergent selection [21] , suggesting that this may be the unit that interacts directly with a cognate ROP5 isoform. Indeed, we were able to demonstrate binding of polymorphic Irgb2 CIM but not Irgb1 CIM to T. gondii virulent strain-derived ROP5B (Fig. 5 ). Two hundred nucleotides in Irgb2 CIM (nt500–nt700) represent a significant hotspot of divergent selection among mouse strains encompassing structural motifs αd and H4. Both αd and H4 constitute essential parts of the polymorphic Irga6 BL/6 interface involved in ROP5 binding [38] , [47] and we could show that these structural elements are also involved in the binding of Irgb2-b1 CIM to ROP5B but not ROP5C. Like Irgb2-b1 BL/6 , the Irgb2-b1 Chimera associated strongly with ROP5C and an Irgb2-b1 CIM ko cell line complemented with Irgb2-b1 Chimera did not confer resistance against T. gondii infection, again indicating a minor role for ROP5C in these T. gondii and mouse strain combinations. T. gondii isolates from South America are genetically highly diverse [4] , [10] , [11] , [12] , [13] , [14] and the majority is associated with high mortality rates in laboratory mice [11] , [15] , and in some cases ROP5 and ROP18 could be demonstrated to be major virulence determinants [50] . Interestingly, all T. gondii strains from South America tested so far are lethal even in CIM mice (Fig. 5 , U. B. Müller and J. C. Howard, unpublished results). To examine the molecular constituents that account for virulence of T. gondii strains from South America in CIM mice, we determined levels of p(T108)Irga6 CIM and Irgb2-b1 CIM at the PVM. In VAND-infected IFNγ-induced CIM cells, the absence of Irgb2-b1 CIM on the vacuole was associated with elevated levels of p(T108)Irga6 CIM . In case of AS28, the Irgb2-b1 CIM loading phenotype was intermediate between RHΔ hxgprt and VAND, but perhaps sufficient to account for the complete absence of Irga6 CIM phosphorylation (Fig. 6a, b ). Consistently, limited binding of AS28-derived ROP5 to Irgb2-b1 CIM could be detected, whereas no interaction with Irgb2-b1 CIM for any of the VAND ROP5 isoforms was visible in our assays (Fig. 6 ). In summary, in VAND infections, escape from Irgb2-b1 CIM binding conclusively results in increased Irga6 CIM phosphorylation and is therefore a very likely explanation for virulence of T. gondii VAND in CIM cells and mice (Fig. 7 ). Decreased vacuolar Irgb2-b1 CIM levels in T. gondii AS28 infections, on the other hand, do not result in increased Irga6 CIM phosphorylation, implicating either different molecular virulence mechanisms not associated with the IRG system or possibly different effector IRG protein targets, not including Irga6. It would appear that the allelic diversity of the tandem IRG protein Irgb2-b1 present in laboratory or some wild-derived strains such as CIM does not include a sequence capable of fully inhibiting the ROP5/ROP18/GRA7 virulence kinase complex of VAND and probably other South American strains. It is interesting to consider whether indeed a suitable Irgb2-b1 allele exists anywhere in the mouse species, and if not, what other, presumably South American, intermediate host species are capable of attenuating the extreme virulence of these T. gondii strains. For the time being, it seems legitimate to consider that the ROP5/ROP18/GRA7 virulence kinase complex is specifically directed against IRG effector proteins. Everything points to accurate molecular complementarity as the basis for the function of the kinase complex, both at the level of the ROP5/IRG interface [38] , [41] , [43] , [47] and the accurate targeting of the rhoptry kinase to the sensitive threonines in the IRG switch region [39] , [40] , [43] . Although GBP have been demonstrated to be associated with resistance to T. gondii in mice [35] , [52] , there is presently no indication that alleles of the ROP5/ROP18/GRA7 system can also be deployed to directly target and phosphorylate this entirely different protein family. Indeed, there is already some evidence that the striking differential virulence of T. gondii strains in mice is not reflected in comparable differences of virulence in humans, where the IRG system has been lost [41] . Lethality of T. gondii for healthy humans is exceedingly rare, and the main differential pathologies seem to be associated primarily with damage to the optic system [54] , [55] . A reasonable hypothesis is that the ROP5/ROP18/GRA7 kinase system has specifically evolved to attenuate an attack by effector proteins of the IRG system on early stages of tachyzoite expansion. The opposed polymorphisms connecting virulence and resistance suggest complex evolutionary dynamics beyond the species level and on a global scale. While it is evident that a big part of the resistance component is due to IRG proteins, it is unlikely that IRG proteins of Mus musculus , an Old World species, are alone responsible for the binding specificities of ROP5 evolved in T. gondii , a parasite almost certainly of New World origin. It is more likely that Irgb2-b1 alleles of evolutionarily significant New World mammals will turn out to be the key resistance factors against New World T. gondii strains. Propagation of T. gondii Tachyzoites of T. gondii strains RHΔ hxgprt [56] , RH-YFP [57] , ME49 [58] , RHΔ rop5 [37] VAND [59] and AS28 [60] were cultivated in confluent monolayers of human foreskin fibroblasts (HS27, ATCC CRL-1634), harvested and immediately used for infection of cells or lysed for subsequent immunoprecipitation or pull-down experiments. Cell culture HEK293T cells (ATTC; CRL-3216) and wt or ko diaphragm-derived cells (DDCs) derived from C57BL/6 and CIM mice [21] were maintained by serial passage in Dulbecco's modified Eagle's medium, high glucose (Invitrogen Life Technologies) supplemented with 2 mM l -glutamine, 1 mM sodium pyruvate, 1× Minimum Essential Medium non-essential amino acids, 100 U ml −1 penicillin, 100 mg ml −1 streptomycin (PAA) and 10% fetal calf serum (FCS, Biochrom). Human foreskin fibroblasts (HS27, ATCC; CRL-1634) were maintained in Iscove's modified Dulbecco's medium, high glucose (Invitrogen Life Technologies) supplemented with 100 U ml −1 penicillin, 100 mg ml −1 streptomycin and 5% FCS. All cells were mycoplasma-free and regularly tested by PCR [61] . Immunological reagents Immunoreagents used in this study were: 3E2 mouse monoclonal antibody against ROP5 isoforms [62] , affinity-purified rabbit sera 87558 against (pT108)Irga6 (1:8000) [39] , 10E7 mouse monoclonal antibody (1:2000) [63] against Irga6, B34 mouse monoclonal antibody (1:2000) [64] against Irgb6, 940/6 rabbit antiserum (1:2000) [43] against Irgb10, 2078 rabbit antiserum (1:1000) [65] against Irgd, 954/1-C15A rabbit antiserum (1:8000 in western blot; 1:4000 in immunofluorescence) [21] against a conserved Irgb-tandem C-terminal peptide, 3.1.2 (1:500) and 2.4.21 (1:1000) rat monoclonal antibodies against T. gondii GRA7 [43] , anti-GST goat antiserum (1:1000 GE Healthcare 27457701), anti-FLAG mouse monoclonal antibody (1:1000, Sigma Aldrich F3165), mouse monoclonal anti-actin antibody (1:1000, Sigma Aldrich A3853) and anti-calnexin rabbit antiserum (1:1000, Merck 208880). Alexa 488 and Alexa 555 labeled donkey anti-rat (A21208) and donkey anti-rabbit (A31572) fluorescent antisera (1:1000, Thermo Fisher Scientific), goat anti-rabbit-HRP (111-035-045), goat anti-rat-HRP (112-035-003), donkey anti-goat-HRP (705-035-147) and rabbit anti-mouse-HRP (315-035-045) (all 1:5000, Jackson Immuno Research Laboratories) polyclonal antibodies were used as secondary reagents. Lysate preparation from free tachyzoites and infected cells The 10–25 × 10 6 free T. gondii tachyzoites or 2.5 × 10 6 DDCs seeded in 10 cm plates were stimulated with 200 U ml −1 IFNγ for 24 h, subsequently infected for 2 h with T. gondii at a multiplicity of infection (MOI) of 10 and washed trifold with phosphate-buffered saline (PBS), and lysed in 800 µl NP-40 lysis buffer (0.1% NP-40, 150 mM NaCl, 20 mM Tris/HCl (pH 7.6), 5 mM MgCl 2 supplemented with protease inhibitors (Roche)) for 2 h under constant rotation at 4 °C. Postnuclear lysates were subjected to immunoprecipitation or pull-down analysis. Immunoprecipitation and pull-down analysis For immunoprecipitation experiments, postnuclear lysates were incubated with the indicated antibodies o/n at 4 °C followed by an additional 1 h of incubation with 100 µl 1:1 (lysis buffer) bead suspension of protein A-Sepharose (Amersham) resin [38] . For pull-down experiments, 100 or 200 pmol (Fig. 3a ) of purified GST or GST-fusion proteins were mixed with 100 µl 1:1 bead suspension of glutathione sepharose 4B (GE Healthcare) resin in 500 µl PBS/2 mM dithiothreitol (DTT) for 1 h at 4 °C. The resin was washed trifold in ice-cold lysis buffer containing 2 mM DTT without detergent and incubated with 800 µl postnuclear T. gondii lysate o/n at 4 °C. Beads were washed trifold with lysis buffer and either stored at −80 °C or immediately boiled in sample buffer (80 mM Tris/HCl (pH 6.8), 5 mM EDTA, 4% SDS, 34% sucrose, 40 mM DTT, 0.002% bromphenol blue) for 5 min at 95 °C and subjected to SDS-PAGE (sodium dodecyl sulfate–polyacrylamide gel electrophoresis) and western blot. Uncropped images of all western blots are provided in the Source Data file. T. gondii replication assay T. gondii proliferation in infected DDCs was determined by incorporation of 3 H-uracil [66] or flow cytometry. For the uracil incorporation assay, cells were grown for 24 h in the presence of IFNγ or left unstimulated, and then infected with T. gondii RH-YFP at different MOIs for an additional 24 h. Cultures were subsequently labeled with 3 H-uracil (0.3 µCi per well) for 24 h, harvested on glass fiber filters and radioactivity incorporated into proliferating T. gondii DNA determined in a beta scintillation spectrometer. For flow cytometry, 1 × 10 5 DDCs seeded in 12-well plates and stimulated with 100 U ml −1 IFNγ for 24 h were infected with RH-YFP. At 24 h post infection, cells were trypsinized, washed 2× with PBS containing 3% FCS (PBS/FCS) and resuspended in 400 µl PBS/FCS containing 1% paraformaldehyde (PFA). After 15 min of incubation at room temperature, fixed cells were washed 2× with PBS/FCS, resuspended in 400 µl PBS/FCS and analyzed by FACSCanto II flow cytometer (BD Biosciences). For each sample, 20,000 events were recorded. Further analysis was performed using FlowJo vX 10.0.7 Software. Percental inhibition of T. gondii replication was defined as follows: 100 − (mean IFNγ-stimulated/mean unstimulated) × 100. Generation of Irgb2-b1 ko cells 2 × 10 5 CIM DDCs were seeded in 6-well plates and cells transfected with CRISPR/Cas9 plasmids (see Plasmid constructs) according to the Lipofectamine 3000 protocol (Invitrogen). At 48 h post transfection, 1 cell per 100 μl was seeded into a well of a 96 - well plate and each well observed for several days to contain only one single colony. Single colonies were transferred to 24-well plates and detergent lysates of IFN-γ-induced (200 U ml −1 ) cells 24 h later analyzed by western blot for Irgb2-b1 CIM expression. Mice virulence assay Female and male mice (25 Mus musculus domesticus , C57BL/6; 44 Mus musculus castaneus , CIM) with ages ranging from 2 to 4 months were infected intraperitoneally with 300 µl or 100 µl of PBS containing freshly harvested tachyzoites of indicated T. gondii strains. Survivors were killed at the indicated days post infection and tested for seroconversion using the Toxocell Latex Kit (Biokit). Data shown are combined from independent experiments. Expression and purification of GST-fusion proteins Recombinant GST-Irgb2-b1 BL/6 , GST-Irgb2-b1 CIM , GST-Irgb2 CIM and GST-Irgb1 CIM proteins were expressed from pGEX-4T-2 constructs in Escherichia coli BL21 after o/n induction with 0.1 mM IPTG (isopropyl β- d -1-thiogalactopyranosid) at 18 °C. Cells were lysed in PBS/2 mM DTT/protease inhibitor (Complete Mini EDTA-free, Roche) using a microfluidiser (EmulsiFlex-C5, Avestin), lysates cleared by centrifugation at 50,000 × g for 60 min at 4 °C and loaded on a GSTrap FF Glutathione Sepharose affinity column (GE Healthcare) in PBS/2 mM DTT. Proteins were eluted with 10 mM reduced l -glutathione in PBS/2 mM DTT and the protein containing fractions subjected to size exclusion chromatography (Superdex 75, Superdex 200; GE Healthcare) [38] . Immunocytochemistry CIM wt and ko DDCs grown on coverslips were infected with T. gondii strains at MOI of 5 for 2 h, washed with PBS, fixed in PBS/4% PFA for 20 min at room temperature and permeabilized in PBS/0.1% saponin for 10 min at room temperature before immunostaining [39] . Microscopy and image analysis was performed blind on coded slides [26] . Intracellular parasites were identified from the pattern of T. gondii GRA7 staining. Yeast two-hybrid assay Saccharomyces cerevisiae strain PJ69-4α was incubated with 1 µg of plasmid DNA (pGAD-C3 or pGBD-C3 containing the indicated genes) in transformation buffer (50% PEG 3350, 0.2 M LiAc, 0.5 mg ml −1 single-stranded DNA, 0.1 M DTT) for 30 min at 42 °C. Cotransformants were selected by plating on double dropout media (SD/-Leu/-Trp). Colonies grown on double dropout media were replica plated again on double dropout media before OD 600 measurement of single colonies resuspended in liquid triple dropout media (SD/-Leu/-Trp/-His). Same amount of material was plated on triple dropout media containing 1 mM 3-AT and incubated for 5 to 10 days at 30 °C. Protein-fragment complementation assay The PCA is based on split TEM - 1 β-lactamase (Bla) of E. coli [67] . Two fragments of the reporter protein (Bla) were fused to two putative interaction partners. The individual Bla fragments are non-functional unless proximity upon interaction of the fused proteins of interest is restored. 7.5 × 10 5 HEK293T cells seeded in 6-well plates were co-transfected with 1 µg respective plasmid DNA using Lipofectamine 3000 reagent following the manufacturer´s instructions (Invitrogen). At 24 h post transfection, cells were trypsinized, washed 1× with PBS and resuspended in 150 µl passive lysis buffer (Promega) containing protease inhibitor cocktail (Roche). After 45 min of incubation on ice and centrifugation for 30 min at 15,000 × g and 4 °C, 50 µl of supernatants were mixed with 15 µl nitrocefin (Abcam), 15 µl H 2 0 and 120 µl PBS in a 96-well plate. The β-lactamase-mediated hydrolysis of nitrocefin was measured by the change of absorbance at 495 nm at intervals of 8–9 s for 50 cycles. In the presence of a standard substrate concentration, the actual nitrocefin hydrolysis rate is dependent on the amounts of reconstituted Bla, consequently on the interaction between the fusion proteins. Therefore, to determine the strength of the interaction, the nitrocefin hydrolysis rates, expressed in mAU min −1 , were calculated for the linear phase of the reaction and compared to each other and the background rates, which were observed upon transfection of the respective fusion proteins alone [67] , [68] . All PCA assays were carried out three times and the differences between average hydrolysis rates were compared to evaluate the strength of the interactions. Plasmid constructs The pGEX-4T-2-Irgb2-b1, pGEX-4T-2-Irgb2 and pGEX-4T-2-Irgb1 constructs allowing expression of recombinant GST-Irgb2-b1, GST-Irgb2 or GST-Irgb1 protein were generated from pGW1H-Irgb2-b1 CIM and pGW1H-Irgb2-b1 BL/6 [21] . Irgb2-b1 CIM, Irgb2-b1 BL/6 and Irgb2-b1 Chimera were amplified from pGEX-4T-2-Irgb2-b1 CIM and pGEX-4T-2-Irgb2-b1 BL/6 and ligated into pGAD-C3, pGBD-C3 and BlaN/BlaC [68] , [69] . The complete coding sequences of VAND rop5 isoforms [41] were subcloned from IDT (Integrated DNA Technologies) vectors into pGAD-C3 and pGBD-C3. VAND gra7 was amplified from T. gondii strain VAND genomic DNA and ligated into pGAD-C3 or pGBD-C3. RH rop5 isoforms were amplified from respective plasmids [43] and ligated into pGAD-C3, pGBD-C3 and BlaN/BlaC. 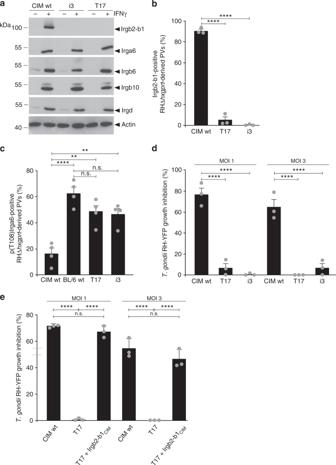Fig. 1 Irgb2-b1CIMis largely responsible for resistance against virulentT. gondiistrains.aWestern blot of detergent lysates from CIM wild-type (wt) andIrgb2-b1CIMknockout (ko) diaphragm-derived cells (DDCs) (T17 and i3) stimulated for 24 h with 200 U ml−1interferon-γ (IFNγ). The signal representing Irgb2-b1CIMin wt cells is lost in both ko cell lines (upper panel). Expression levels of all other Immunity-Related GTPases (IRG) proteins are unchanged in ko cell lines compared with wt cells (middle panels). Actin serves as loading control (lower panel).b,cFrequency of vacuoles positive for Irgb2-b1CIM(b) or Irga6CIMphosphorylated at T108 p(T108)Irga6CIM) (c) detected by immunofluorescence with anti-p(T108)Irga6CIMor anti-Irgb2-b1CIMantibodies in IFNγ-induced (200 U ml−1) wt CIM and BL/6 orIrgb2-b1CIMko CIM DDCs infected for 2 h with RHΔhxgprt. Error bars indicate the mean and standard error of the mean (SEM) of three (b) or four (c) independent experiments (about 100 vacuoles were counted per experiment). One-way analysis of variance (ANOVA) followed by Tukey's multiple comparison was used to test differences between groups; ****p< 0.0001; **p< 0.0025; n.s. not significant.bNo Irgb2-b1CIMpositive vacuoles were found inIrgb2-b1CIMko cells.cFrequencies of p(T108)Irga6CIM-positive vacuoles in ko cells are significantly increased in comparison with wt cells.d,eCIM DDCs were induced with 100 U ml−1IFNγ for 24 h and infected withT. gondiiRH-YFP at a multiplicity of infection (MOI) of 1 or 3. Intracellular parasite growth was determined by flow cytometry 24 h post infection as described in Methods. Error bars indicate the mean and SEM of three independent experiments. One-way ANOVA followed by Tukey's multiple comparison was used to test differences between groups; ****p< 0.0001; n.s. not significant.dControl ofT. gondiireplication is lost in wt BL/6 andIrgb2-b1CIMko CIM DDCs compared with wt CIM DDCs.eControl ofT. gondiireplication is restored to wt levels (wt CIM DDCs) inIrgb2-b1CIMko CIM DDCs complemented withIrgb2-b1CIM(T17+Irgb2-b1CIM) A complete list of primers is given in Supplementary Table 1 . The pGBD-C3-ROP18 construct was generated earlier [39] . The following gRNAs were hybridized with their complementary strand and cloned into pX335 (Addgene) at the CACCG insertion site to generate Irgb2-b1 CIM ko constructs: Irgb2-b1 1: 5'-caccgTGGGTATGATTTTTTCTCAA-3' Irgb2-b1 2: 5'-caccgGTTGTATATACCACCCCAAC-3'. Lentiviral transduction Lentiviral transduction was applied to generate Irgb2-b1 CIM ko cells overexpressing Irgb2-b1 variants. For this purpose, gag - pol -expressing and env -expressing plasmids were co-transfected with the plasmid carrying the gene of interest into HEK293T cells that have been grow to a density of 70% in a 10 cm plate. At 24 h post transfection, the medium was exchanged and cells incubated for additional 24 h. The supernatant was filtered and transferred to Irgb2-b1 CIM ko cells (T17) that have been seeded 1 day before in a 6 cm plate and grown to a density of 70%. After 24 h, cells were harvested and transferred into appropriate cells culture flasks with medium containing 1–5 µg ml −1 puromycin for selection of transduced cells. Statistics All statistical analyses were performed using GraphPad Prism 7.0 software (GraphPad). P values were determined by an appropriate statistical test. Statistical differences in IRG protein intensities between groups at single T. gondii -derived intracellular vacuoles were determined using a two-tailed Student’s t -test. One-way analysis of variance (ANOVA) followed by Tukey's multiple comparisons or Kruskal–Wallis test followed by Dunn's multiple comparisons were used to test differences in IRG protein frequencies or intensities between more than two groups at T. gondii -derived intracellular vacuoles respectively. Statistical differences for T. gondii replication analyzed by FACS were determined using one-way ANOVA followed by Tukey's or Dunnett's multiple comparisons. In case of PCA assays, one-way ANOVA followed by Tukey's multiple comparison was used to test differences between groups. 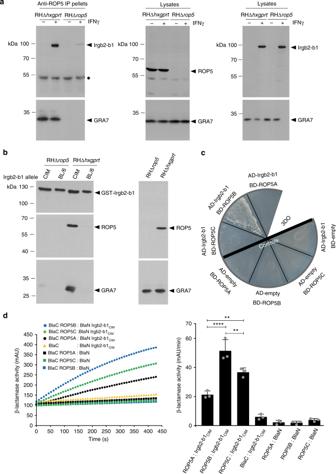Fig. 2 Irgb2-b1CIMdirectly bindsT. gondii-derived ROP5B and ROP5C.aIrgb2-b1CIMwas co-imunoprecipitated from RHΔhxgprt- but not RHΔrop5-infected CIM diaphragm-derived cells (DDCs) that have been induced with 200 U ml−1interferon-γ (IFNγ) using a ROP5-specific antibody (upper left hand panel). The lower left hand panel indicates GRA7 association with ROP5 immunoprecipitations. The star indicates a protein unspecifically detected by the antibody used for immunoprecipitation. The middle and right hand panels display amounts of ROP5, GRA7 and Irgb2-b1 in the lysates used for immunoprecipitation.bPull-down of ROP5 by CIM but not BL/6 GST-Irgb2-b1 from RHΔhxgprtdetergent lysates. RHΔrop5tachyzoite detergent lysates have been included as control (middle left hand panel). The lower panel indicates GRA7 association with ROP5. The upper panel indicates input of glutathioneS-transferase (GST)-fusion proteins in the pull-down. The right hand blot shows ROP5 (upper panel) and GRA7 (lower panel) levels in tachyzoite lysates.cIrgb2-b1CIMinteracts with ROP5B and ROP5C but not ROP5A in a yeast two-hybrid approach. Proteins were expressed either as fusion to a transcriptional activation domain (AD) from pGAD-C3 or to a DNA-binding domain (BD) from pGBD-C3. Colony growth under 3DO conditions is indicative of protein/protein interaction. The bold black line separates samples from negative controls.dProtein-fragment complementation assay. Proteins were fused to N-terminal (BlaN) or C-terminal (BlaC) fragments of the reporter proteinTEM-1β-lactamase. The increase in absorbance measured at 405 nm indicates restoration of β-lactamase activity after protein/protein interaction. Binding of Irgb2-b1CIMto ROP5B is significantly stronger compared to ROP5C and ROP5A. Error bars indicate the mean and standard deviation of three independent experiments (right hand panel). One-way analysis of variance (ANOVA) followed by Tukey's multiple comparison was used to test differences between groups; ****p< 0.0001; **p< 0.0025. The kinetic of the β-lactamase reaction is shown for one representative experiment (left hand panel) All error bars indicate the mean and standard error of the mean (SEM) or standard deviation of at least three independent experiments. The p values < 0.05 were considered to be significant. 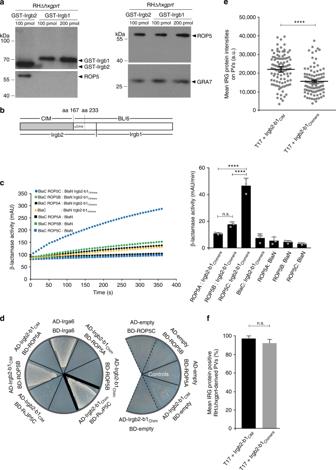Fig. 3 The Irgb2-b1CIMinterface forT. gondiiROP5B binding is polymorphic.aPull-down ofT. gondiiROP5 by GST-Irgb2CIMbut not GST-Irgb1CIMfrom RHΔhxgprttachyzoite detergent lysates (lower left hand panel). The upper left hand panel indicates input of glutathioneS-transferase (GST)-fusion proteins in the pull-down. The right hand panels display amounts of ROP5 (upper panel) and GRA7 (lower panel) in the tachyzoite lysate used for the pull-down.bSchematic representation of Irgb2-b1 CIM-BL/6 chimeric variant (Irgb2-b1Chimera) used in (c,d).c,dIrgb2-b1CIMinteraction withT. gondiiROP5B but not ROP5C is disturbed in case of Irgb2-b1Chimera.cProtein-fragment complementation assay. Proteins were fused to N-terminal (BlaN) or C-terminal (BlaC) fragments of the reporter proteinTEM-1β-lactamase. Error bars indicate the mean and standard deviation of three independent experiments (right hand panel). One-way analysis of variance (ANOVA) followed by Tukey's multiple comparison was used to test differences between groups; ****p< 0.0001; n.s. not significant. The kinetic of the β-lactamase reaction is shown for one representative experiment (left hand panel). Interaction of Irgb2-b1CIMwithT. gondiiROP5B is almost completely abrogated with Irgb2-b1Chimera.dYeast two-hybrid approach. Proteins were expressed either as fusion to a transcriptional activation domain (AD) from pGAD-C3 or to a DNA-binding domain (BD) from pGBD-C3. Colony growth under 3DO conditions is indicative of protein/protein interaction. Black dotted lines indicate assembly of relevant areas from two different plates.eIntensities of individual vacuoles positive for Irgb2-b1CIMand Irgb2-b1Chimeradetected by immunofluorescence with anti-Irgb2-b1-specific antiserum in interferon-γ (IFNγ)-induced (200 U ml−1) wild-type (wt) CIM diaphragm-derived cells (DDCs) infected for 2 h with RHΔhxgprt. Intensities of Irgb2-b1Chimeraare significantly reduced at RHΔhxgprt-derived vacuoles.fFrequency of Irgb2-b1CIM- and Irgb2-b1Chimera-positive vacuoles detected by immunofluorescence with anti-Irgb2-b1-specific antiserum in IFNγ-induced (200 U ml−1) complementedIrgb2-b1ko CIM DDCs infected for 2 h with RHΔhxgprt(about 100 vacuoles were counted per experiment). No differences in numbers of Irgb2-b1CIM- and Irgb2-b1Chimera-positive vacuoles could be observed. Ineandf, error bars indicate the mean and SEM of three independent experiments. Student's t-test was used for two-group comparisons; ****p< 0.0001, n.s. not significant 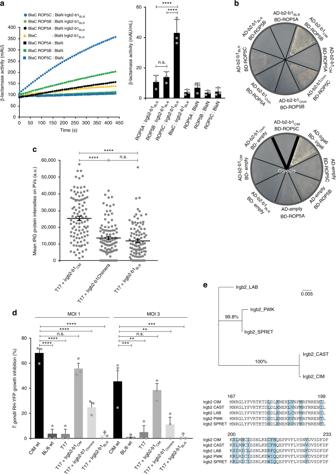Fig. 4 Irgb2-b1BL/6directly binds ROP5C.aProtein-fragment complementation assay. Proteins were fused to N-terminal (BlaN) or C-terminal (BlaC) fragments ofTEM-1β-lactamase. One-way analysis of variance (ANOVA) followed by Tukey's multiple comparison was used to test differences between groups; ****p< 0.0001; n.s. not significant. The kinetic of the reaction is shown for one representative experiment (left hand panel). Irgb2-b1BL/6interacts withT. gondiiROP5C but not ROP5B and ROP5A.bYeast two-hybrid. Proteins were expressed as fusion with transcriptional activation domain (AD) from pGAD-C3 or DNA-binding domain (BD) from pGBD-C3. Colony growth is indicative of Irgb2-b1BL/6and Irgb2-b1Chimerainteraction with ROP5C and Irgb2-b1CIMinteraction with ROP5B. Bold black lines separate samples from negative controls.cIntensities of individual vacuoles detected by immunofluorescence with anti-Irgb2-b1-specific antiserum in interferon-γ (IFNγ)-induced (200 U ml−1) cells infected for 2 h with RHΔhxgprt. Kruskal–Wallis test followed by Dunn's multiple comparisons was used to test differences between groups; ****p< 0.0001; n.s. not significant. Intensities of Irgb2-b1BL/6and Irgb2-b1Chimeraare reduced at RHΔhxgprt-derived vacuoles.dPolymorphic Irgb2-b1CIMinterface mediating ROP5B binding is crucial forT. gondiicontrol in vitro. CIM diaphragm-derived cells (DDCs) were induced with 100 U ml−1IFNγ for 24 h and infected withT. gondiiRH-YFP at a multiplicity of infection (MOI) of 1 or 3. Parasite growth was determined by flow cytometry 24 h post infection. One-way ANOVA followed by Dunnett's multiple comparisons was used to test differences between CIM wild-type (wt) and other cells; ****p< 0.0001; ***p< 0.0008; **p< 0.006; n.s. not significant. Control ofT. gondiivirulent strain replication is lost inIrgb2-b1CIMko CIM DDCs complemented withIrgb2-b1Chimera.eUpper panel, phylogenetic analysis and maximum likelihood tree ofIrgb2sequences (CIM,M. m. castaneus; CAST,M. m. castaneus; LAB,M. m. domesticus; PWK,M. m. musculus; SPRET,Mus spretus). LAB indicates the allele shared by all laboratory mice tested so far, including C57BL/621. Only bootstrap values above 50 are shown. Lower panel, alignment of Irgb2 amino acids M167 to P233 encompassing putative structural motifs αd and H4. Polymorphic sites are highlighted in blue. Error bars indicate the mean and SEM or standard deviation of three independent experiments 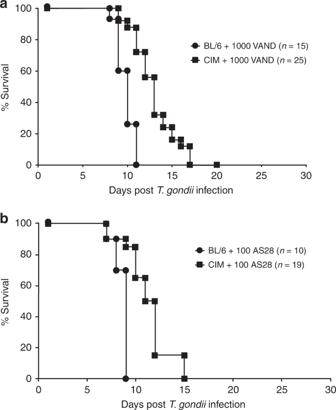Fig. 5 South AmericanT. gondiiVAND and AS28 evade growth restriction in CIM mice. CIM wild-type (wt) (a,n= 25;b,n= 19) and C57BL/6 (a,n= 15;b,n= 10) mice were infected by intraperitoneal injection of 1000T. gondiiVAND (a) or 100 AS28 (b) strain parasites and survival monitored for 15–20 days. Data shown are combined from three (a) or two (b) independent experiments Ethics statement All experiments with mice at the University of Cologne were conducted under the regulations and protocols for animal experimentation in accordance with guidelines of the European Commisson (Directive 2010/63/EU) and approved by the local government authorities (Bezirksregierung Köln, Germany), LANUV Nordrhein-Westfalen Permit No. 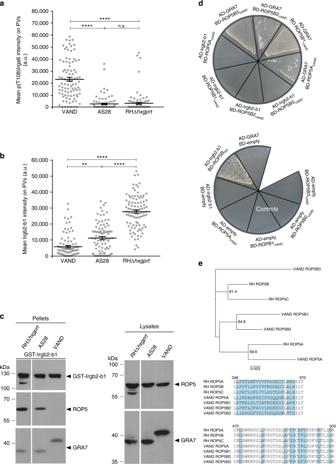Fig. 6 T. gondiiVAND-derived ROP5 escapes targeting by Irgb2-b1CIM.ap(T108)Irga6CIMprotein intensities are increased at VAND-derived vacuoles. interferon-γ (IFNγ)-induced CIM diaphragm-derived cells (DDCs; 200 U ml−1) were infected for 2 h with indicatedT. gondiistrains and individual p(T108)Irga6CIM-positive vacuoles identified with 558 p(T108)Irga6CIM-specific antiserum. Error bars indicate the mean and SEM of three independent experiments. Kruskal–Wallis test followed by Dunn's multiple comparisons was used to test differences between groups; ****p< 0.0001; n.s. not significant.bIrgb2-b1CIMintensities are reduced at VAND- and AS28-derived vacuoles. IFNγ-induced CIM DDCs (200 U ml−1) were infected for 2 h with indicatedT. gondiistrains and individual Irgb2-b1CIM-positive vacuoles identified with anti-Irgb2-b1-specific antiserum. Error bars indicate the mean and SEM of three independent experiments. Kruskal–Wallis test followed by Dunn's multiple comparisons was used to test differences between groups; ****p< 0.0001; **p< 0.006.cIn vitro pull-down with recombinant GST-Irgb2-b1CIMfusion protein andT. gondiitachyzoite detergent lysates. Pull-down of ROP5 by Irgb2-b1CIMis reduced with AS28 and completely lost in case of VAND tachyzoite lysates compared to RHΔhxgprt-derived ROP5 (middle left hand panel). VAND GRA7 pull-down is not dependent on ROP5 (lower panel). The upper panel indicates input of GST-Irgb2-b1CIMin the pull-down. The right hand blot shows ROP5 (upper panel) and GRA7 (lower panel) levels in tachyzoite lysates. All tracks were run on a single gel; vertical white lines indicate excision of irrelevant tracks.dVAND ROP5 isoforms ROP5A, ROP5B1, ROP5B2 and ROP5B3 do not directly interact with Irgb2-b1CIMor VAND GRA7 in a yeast two-hybrid approach. Proteins were expressed either as fusion to a transcriptional activation domain (AD) from pGAD-C3 or to a DNA-binding domain (BD) from pGBD-C3. Colony growth under 3DO conditions is indicative of protein/protein interaction. Bold black line separates samples from negative controls.eUpper panel, alignment ofT. gondiiRH and VAND ROP5 amino acid sequences that represent a polymorphic hotspot and have been shown to be involved in binding to Irga6BL/6. Polymorphic sites are highlighted in blue. Lower panel, phylogenetic analysis and maximum likelihood tree ofT. gondiiRH and VANDrop5sequences. Only maximum likelihood bootstrap values above 50 are shown 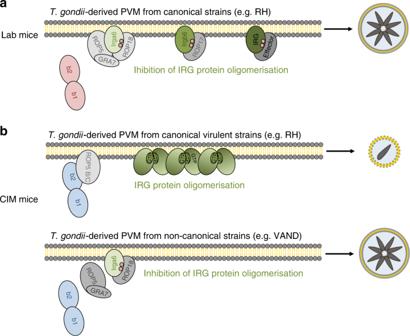Fig. 7 Model for Irgb2-b1-mediated control ofT. gondiiinfection in wild-derived mice.aIn laboratory mice, effector proteins from canonical virulentT. gondiistrains (like RH) specifically phosphorylate certain Immunity-Related GTPases (IRG) proteins, thereby inhibiting oligomerisation and destruction of the parasitophorous vacuolar membrane (PVM). Two rhoptry kinases, ROP18 and ROP17, have been demonstrated to preferentially phosphorylate Irga6BL/6or Irgb6BL/6. The existence of additional parasite effectors specific for other IRG proteins is assumed.bIn CIM and probably other wild-derived mice, canonical virulentT. gondiistrains (like RH) are counteracted by direct binding of ROP5 isoform B by the polymorphic tandem IRG protein Irgb2-b1CIM. IRG effector proteins are free to accumulate around the PVM, resulting in growth control, encystment and transmission of the parasite. Genetically more diverseT. gondiistrains, likeT. gondiiVAND from South America, express polymorphic ROP5 variants that are not targeted by Irgb2-b1CIM. Consequently, effector IRG proteins such as Irga6CIMare phosphorylated and inactivated by aT. gondiiVAND kinase complex. Infected animals die shortly after parasite challenge. Molecular interaction between ROP18 and ROP5 or Irga6 and ROP5 within the VAND kinase complex awaits experimental confirmation 44.07.189. Procedures using live animals at Instituto Gulbenkian de Ciência were approved by the Instituto Gulbenkian de Ciência ethical committee and by the national animal welfare authority (DGAV) and were carried out in accordance with national (portaria 1005/92) and European (Directive 56/609/CE) regulations Reporting summary Further information on experimental design is available in the Nature Research Reporting Summary linked to this article.